Ultrahigh-capacity non-periodic photon sieves operating in visible light Miniaturization of optical structures makes it possible to control light at the nanoscale, but on the other hand it imposes a challenge of accurately handling numerous unit elements in a miniaturized device with aperiodic and random arrangements. Here, we report both the new analytical model and experimental demonstration of the photon sieves with ultrahigh-capacity of subwavelength holes (over 34 thousands) arranged in two different structural orders of randomness and aperiodicity. The random photon sieve produces a uniform optical hologram with high diffraction efficiency and free from twin images that are usually seen in conventional holography, while the aperiodic photon sieve manifests sub-diffraction-limit focusing in air. A hybrid approach is developed to make the design of random and aperiodic photon sieve viable for high-accuracy control of the amplitude, phase and polarization of visible light. The polarization independence of the photon sieve will also greatly benefit its applications in optical imaging and spectroscopy. Nanotechnology has provided a strong support for realizing the goal of controlling light at the nanoscale by using various nanostructures. This enabled the emergence of new physical phenomena, such as surface-enhanced Raman scattering [1] , extraordinary optical transmission [2] , [3] and surface plasmons optics [4] . However, miniaturization of structures gives rise to an intractable problem particularly for controlling visible light with devices composed of enormous unit elements, that is, realization of superfocusing in air by beating the diffraction limit beyond the evanescent range [5] . Creation of a small focusing spot necessitates high spatial frequency to be carried by the transmitted beam [5] , which imposes inseparable conditions for a large array size and a huge number of unit elements. Recently, devices with aperiodic or randomly distributed nanostructures have drawn great attention [6] owing to their novel properties, such as absorption-enhancing proximity effect [7] and near-field manipulation of light [8] . Nanophotonic devices can acquire rich degrees of freedom (that is, spatial position and geometric size of the nanostructure) from structural aperiodicity and randomness to realize complex functionalities, which are not achievable through periodic or quasi-periodic features with limited control in geometry [9] , [10] . However, the physics of designing such a kind of aperiodic or random device possessing a large capacity of both position-/size-varying unit structures are yet to be explicitly addressed upon technical challenges. The first challenge comes from the lack of an effective strategy to determine the geometry positions and sizes of individual holes, in particular for the aperiodic and random cases. The second challenge lies in the unavailability of an appropriate method for direct modelling of the overall device performance oriented by specific objectives such as holography-based beam shaping with high uniformity and superfocusing, which require highly accurate information about the optical field diffracted from an individual nanostructure. One approach reported recently was to approximate the optical performance (that is, amplitude and phase of diffracting light) of a single nanostructure by using that of its periodic array [11] . Owing to inadequate accuracy, this method only worked well in paraxial optics for conceptual demonstration of optical holography [12] , [13] and optical focusing without breaking the diffraction limit [14] , [15] , [16] , [17] . To overcome these challenges, we propose a hybrid approach that strategically combines the coupled-mode theory and the multipole expansion method to describe the diffracted field from a huge number of subwavelength holes with high accuracy. It gains physical insight into the diffraction issue in terms of elementary mathematical functions, and it makes the optimization algorithms feasible in the structural design of a photon sieve aiming for high-quality holograms and superfocusing. Having validated it experimentally, we report a random photon sieve composed of 34,034 subwavelength holes, demonstrating an optical hologram with a diffraction efficiency of 47%, as well as high uniformity along with polarization independence. To show its high accuracy for spatial light manipulation, another photon sieve consisting of 7,240 size-varying subwavelength holes, aperiodically located at 22 concentric rings, is used to experimentally realize a sub-diffraction-limit focal spot with a full width at half maximum (FWHM) of ∼ 0.32 λ in air (instead of dielectric media [18] or photoresist [19] ), which is formed at a distance of about 21 λ away from the aperture under visible-light illumination ( λ =632.8 nm). This work offers a viable method to tackle ultrahigh-capacity random or aperiodic subwavelength features to accurately tailor the functionalities of optical devices via manipulating phase, amplitude and polarization of light beyond the evanescent region. Hybrid approach Although the vectorial Rayleigh–Sommerfeld diffraction and angular spectrum theory have been proposed to carry out the simulation of diffraction field at a targeted plane of photon sieves [9] , [10] , [20] , lack of essential capacity in describing the polarization and intensity profiles of electric field immediately after a single nanohole makes them behave inaccurately for far-field diffraction. Succeeding in it as a powerful tool [21] , finite-difference time domain (FDTD) demands tremendous computing resources to create ultrafine grids so as to accurately calculate the vector field in overall space, not to mention the huge degree of uncertainties during the optimization of such a complex photon sieve. To alleviate this issue, we propose a twofold method: (1) a hybrid approach combining the coupled-mode theory [3] , [22] and multipole expansion method [23] , [24] is proposed to accurately model the optical field diffracted from one single subwavelength hole, as shown in Fig. 1a , which is formulated by the superimposing elementary mathematical functions (see equation (3) in the Methods section); (2) the far-field diffracted field of the entire photon sieve sketched in Fig. 1b is obtained by coherently superimposing optical fields diffracted from each subwavelength hole (see equation (4)). A comparison between our method and FDTD for calculating a relatively small photon sieve has been carried out with good agreement, as detailed in the Supplementary Figs 1–4 and Supplementary Notes 1–4 . It verifies the effectiveness and reliability of this hybrid approach. In our method, the size parameter (that is, radius a ) and position information of the subwavelength hole are taken into account to get its diffraction characteristics by calculating the electric field of interest only, which is free from the requirement of simulating the electric field in the whole space by FDTD. This hybrid approach greatly improves the efficiency in optimizing the design in terms of arbitrary distribution, size variation and boundless number. 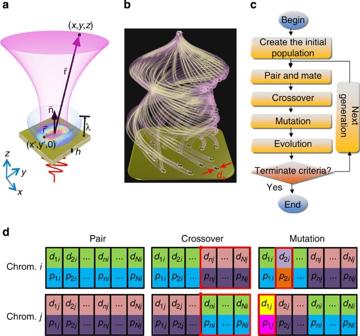Figure 1: Concept of photon sieve and its hybrid design approach. (a) Far-field diffraction of light from a unit hole perforated on a perfect-electric-conductor film with a thickness ofh. Evanescent wave confined in one wavelength (λ) has no contribution to the far-field diffraction.is the position vector at the exit plane of the hole,is the external normal vector andis spatial vector of a view point (x,y,z). (b) Sketch of controlling light beyond the evanescent region by a photon sieve. Every nanohole works as a single diffraction unit, and their interference pattern can be controlled by hole position and sizedn. (c) Flowchart of standard genetic algorithm containing the pair, cross-over and mutation operations. (d) Sketch of cross-over and mutation operation between two paired chromosomes that encode the hole sizednand postionpn(n=1, 2, …,N) of the photon sieve. Figure 1: Concept of photon sieve and its hybrid design approach. ( a ) Far-field diffraction of light from a unit hole perforated on a perfect-electric-conductor film with a thickness of h . Evanescent wave confined in one wavelength ( λ ) has no contribution to the far-field diffraction. is the position vector at the exit plane of the hole, is the external normal vector and is spatial vector of a view point ( x , y , z ). ( b ) Sketch of controlling light beyond the evanescent region by a photon sieve. Every nanohole works as a single diffraction unit, and their interference pattern can be controlled by hole position and size d n . ( c ) Flowchart of standard genetic algorithm containing the pair, cross-over and mutation operations. ( d ) Sketch of cross-over and mutation operation between two paired chromosomes that encode the hole size d n and postion p n ( n =1, 2, …, N ) of the photon sieve. Full size image Design principle Genetic algorithm inspired by biological evolution [25] is used to implement the design, because it can be easily combined with other algorithms such as particle swarm optimization [26] , cuckoo search [27] and ant colony optimization [28] owing to their common inheritance on old generation. The basic configuration containing key operations of pair, cross-over and mutation are schematically shown in Fig. 1c . After the standard genetic algorithm, we encode the photon sieve information into one chromosome containing N genes, each of which is labelled by the hole size ( d n ) and position ( p n ), as shown in Fig. 1d . The evolution operation of every chromosome can thus be carried out on the basis of the hybrid approach. In practice, the hole size is constrained to a certain range owing to fabrication issues, which implies that we only need to calculate the electric field of light diffracted from some limited-geometry holes before the evolution operation. Next, we superimpose the known electric field of every hole by addressing its size. It significantly expedites an evolution operation by four orders of magnitude (see Supplementary Fig. 5 and Supplementary Notes 5–6 ), which makes it more feasible in carrying out the design of a large-scale photon sieve. Optical hologram A randomly distributed photon sieve to realize high-uniformity optical holography is schematically shown in Fig. 2a . The design of the photon sieve is implemented by a modified genetic algorithm with mutation and evolution operations only (see Supplementary Fig. 5 and Supplementary Note 6 ). The photon sieve was fabricated with 34,034 holes of 150 nm radius randomly distributed in a 100-nm-thick chromium film via electron-beam lithography (ELS-7000, Elionix). The scanning electron microscope images, as depicted in the inset, clearly show randomness with the minimum center-to-center distance of 450 nm between two neighbouring holes, which demonstrates an improvement by nearly 200 times in spatial resolution than the similar halftone-based hologram with the smallest pixel pitch of 80 μm [29] , [30] , [31] . 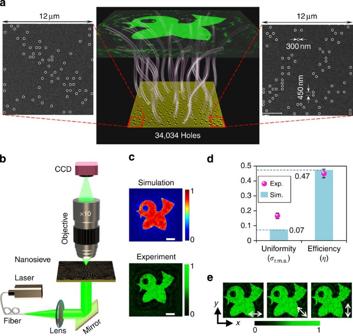Figure 2: Random photon sieve for an optical hologram. (a) Sketch of photon sieve hologram (149 × 149 μm) with a target plane located 500 μm away from its surface. Insets: scanning electron microscope images of the left and right bottom of the photon sieve. (b) Experimental setup for optical holography characterization. (c) Simulated and measured intensity profiles with a bird pattern. Scale bar, 30 μm. (d) Quality evaluation of a photon sieve hologram by using its uniformity (σr.m.s.) and diffraction efficiency (η) with simulated (histograms) and experimental (dots) data. (e) Experimental verification of incidence polarization independence of the photon sieve hologram. White double arrows show the incidence polarization directions (0°, 45° and 90°). Figure 2: Random photon sieve for an optical hologram. ( a ) Sketch of photon sieve hologram (149 × 149 μm) with a target plane located 500 μm away from its surface. Insets: scanning electron microscope images of the left and right bottom of the photon sieve. ( b ) Experimental setup for optical holography characterization. ( c ) Simulated and measured intensity profiles with a bird pattern. Scale bar, 30 μm. ( d ) Quality evaluation of a photon sieve hologram by using its uniformity ( σ r.m.s. ) and diffraction efficiency ( η ) with simulated (histograms) and experimental (dots) data. ( e ) Experimental verification of incidence polarization independence of the photon sieve hologram. White double arrows show the incidence polarization directions (0°, 45° and 90°). Full size image We experimentally verified the performance of this photon sieve by normally projecting a linearly polarized 532-nm-wavelength light on it and collecting the transmitted light with a × 10 magnification objective lens. The intensity was directly recorded by a charge-coupled device camera, as shown in Fig. 2b . A bird pattern is identically reconstructed by the simulated and measured intensity profiles, as shown in Fig. 2c with excellent agreement. The intensity uniformity is defined as σ r.m.s. =[<( I ( x , y )− Ī ) 2 >/ Ī 2 ] 1/2 , where I ( x , y ) denotes the intensity inside the bird pattern area, Ī =< I ( x , y )> and <·> stands for the average intensity and the average operator, respectively. The simulated σ r.m.s. equals 7%, which is so small that it even behaves better than traditional holography for beam shaping (for example, ∼ 11% in ref. 32 ). As shown in Fig. 2d , the measured σ r.m.s. shows a uniformity of ∼ 17%, which might attribute to the imperfection (for example, irregularly circular shape, the hole's in-wall not perpendicular to the exit surface) of fabricated holes. The dependence of the uniformity on the incident wavelength (ranging from 460 to 580 nm) has been simulated. Our results (not shown here) demonstrate that the amplitude uniformity varies within less than 1% in the aforementioned wavelength range. We have also investigated the diffraction efficiency formulated by η = I t / I 0 , where I t is the total intensity of the bird pattern and I 0 is the transmitted intensity. Both of the simulated and measured results have an approximately equal value of ∼ 47%, as shown in Fig. 2d . This means that nearly half of the transmitted intensity contributes to the reconstruction of the image. It is a significant advantage over metasurface holograms with polarization dependence [12] , [13] , because half of their transmitted light is filtered out by a polarizer. That, in fact, leads to much lower diffraction efficiency (below 20% in refs 12 , 13 , 32 , 33 , 34 , 35 ). Owing to the rotational symmetry of the circular hole, our photon sieve hologram exhibits overall polarization independence to account for high diffraction efficiency. Plotted in Fig. 2e are the experimentally captured images of nearly identical intensity profiles when varying the polarization orientation of incident light at 0°, 45° and 90° (angle between the x axis and polarization), respectively. Beyond these, our photon sieve hologram is free from problematic twin image and high-order diffraction that are present in nanostructured- [33] , [34] , nanotube- [35] and nanoparticle-based [36] holograms. Traditionally, the twin image also appears for spatial light modulators, and it has been the subject of a long-standing debate [37] , [38] , [39] , [40] since holography was invented in 1948 ref. 41 . Our results suggest that the twin image could be eliminated when the size of the elementary diffraction unit (DU) of the hologram is chosen to be smaller than the wavelength, as demonstrated in refs 12 , 13 . In our case, this DU is a 150-nm-radius hole purposely made at the subwavelength scale, whereas the elementary DU (consisting of several pixel pitches) of those nanostructured holograms [33] , [34] is larger than the wavelength. For nanotube- [35] and nanoparticle-based [36] holograms with twin images, their effective DUs with a wavelength-scale size can be taken as a combination of two horizontally or vertically pixel pitches, because two neighbouring pixel pitches share the same phase or amplitude in the hologram design. In their design processes, the retrieval of phase or amplitude in a hologram is based on the feedback of optical inverse fast Fourier transform of target intensity, which has no capacity to distinguish the high spatial frequency embedded in two subwavelength pixels (in connection with evanescent wave), resulting in an effective DU larger than the wavelength. To avoid this in designing the photon sieve hologram, we used the genetic algorithm based on our hybrid approach and made an exemplary attempt by randomly addressing the isolated nanoholes in hologram without referring to the amplitude or phase feedback [35] , [36] , which has followed the proposal by Gerchberg and Saxton [42] . Superfocusing Far-field super-resolution focusing under visible light has been demonstrated with periodically or quasi-periodically structured lenses [9] , [10] . The requirements on a large amount of nanostructures and accurate manipulation of light beyond the evanescent region are challenging in simulation and design optimization. As a result, most approaches adopt the lens with its nanostructures arranged in period or quasi-period distribution having limited manipulation of light. To obtain a circular focusing spot, we propose an optical nanosieve with circular symmetry as sketched in Fig. 3a , composed of 7,240 subwavelength holes located at 22 concentric rings with a radius of R n ( n is the index of rings with an ascending order from inner to outer). These rings are non-periodically distributed in radial position, while the holes in each ring are uniformly allocated and equally sized with a radius of a n . When n increases, a n reduces from 150 nm ( n =1) to 50 nm ( n =22), while R n rises from 10.85 to 19.65 μm. Hence, the overall structure exhibits aperiodic behaviour in a n and R n , which allows it to sieve light with appropriate amplitude and phase for achieving a small spot [43] . The central region blocks the direct transmission of light carrying low spatial frequencies while only the component of high spatial frequencies passes through to constructively interfere, accounting for a sharp focusing [5] . The correlation between a n and R n can be encoded by the hole diameter d n and the interval t n between adjacent rings. The parameters d n and t n are used to construct the chromosome information, which could be systematically optimized (see Supplementary Fig. 7 and Supplementary Note 7 ) through the standard genetic algorithm to reach a sub-diffraction-limit focusing spot. 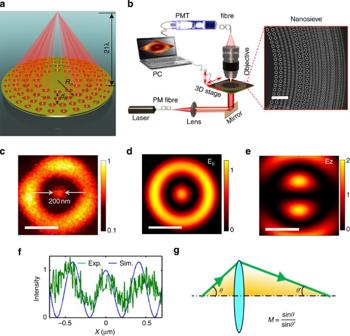Figure 3: Aperiodic photon sieve for superfocusing. (a) Sketch of a photon sieve composed of 22 non-periodically arrayed concentric annuli.Rnis the radius of thenth ring with identical holes havingdnin diameter. (b) Measurement setup and scanning electron microscope image of a part of the fabricated photon sieve. PC, personal computer; PMT, photomultiplier tube. Scale bar, 2 μm. (c) Measured spot of 200 nm at the target plane, which is about 21λaway from the surface under 632.8-nm-wavelength illumination. Scale bar, 500 nm. (d) Intensity profile of transversely polarized fieldE||(=Exex+Eyey). It is normalized to the peak intensity of the central spot (x=0 andy=0). Scale bar, 500 nm. (e) Intensity profiles of longitudinal fieldEz. Its intensity is normalized to the peak intensity of central transversely polarized spot ind. Scale bar, 500 nm. (f) Cross-sectional intensity profiles of the experimental result (green) incand the theoretical result (blue) ind. (g) Sketch of an objective lens with a magnification ofM, corresponding to the attenuation ofEzat the imaging plane. Figure 3: Aperiodic photon sieve for superfocusing. ( a ) Sketch of a photon sieve composed of 22 non-periodically arrayed concentric annuli. R n is the radius of the n th ring with identical holes having d n in diameter. ( b ) Measurement setup and scanning electron microscope image of a part of the fabricated photon sieve. PC, personal computer; PMT, photomultiplier tube. Scale bar, 2 μm. ( c ) Measured spot of 200 nm at the target plane, which is about 21 λ away from the surface under 632.8-nm-wavelength illumination. Scale bar, 500 nm. ( d ) Intensity profile of transversely polarized field E || (=E x e x +E y e y ). It is normalized to the peak intensity of the central spot ( x =0 and y =0). Scale bar, 500 nm. ( e ) Intensity profiles of longitudinal field E z . Its intensity is normalized to the peak intensity of central transversely polarized spot in d . Scale bar, 500 nm. ( f ) Cross-sectional intensity profiles of the experimental result (green) in c and the theoretical result (blue) in d . ( g ) Sketch of an objective lens with a magnification of M , corresponding to the attenuation of E z at the imaging plane. Full size image Figure 3b depicts the measurement setup with an illumination wavelength of 632.8 nm, and the inset shows the scanning electron microscope image of a part of the fabricated aperiodic photon sieve (the structural dimensions and fabrication process are provided in detail in Supplementary Table 1 and Supplementary Notes 8 and 9 ). Figure 3c shows the experimentally scanned intensity pattern at the focal plane in an area of 1.2 × 1.2 μm with a step size of 6 nm. A sub-diffraction-limit focal spot with about 200-nm FWHM (≈0.32 λ ) is formed at a distance of z =13.3 μm (≈21 λ at λ =632.8 nm) together with an annular side lobe. Figure 3d correspondingly plots the theoretical intensity profile of transversely polarized field E || . The agreement between the experimental spot and theoretical E || indicates that the recorded focal spot is transversely polarized, while the longitudinal component E z predicted in Fig. 3e becomes experimentally undetectable. Furthermore, we plot the normalized cross-sectional profiles of experimental and theoretical results in Fig. 3f without any fitting, and both match with each other with a small discrepancy of amplitude and lateral position, which can be attributed to the cumulative error of the three-dimensional stage and the imperfect alignment between photon sieve and objective lens. The experimental absence of a longitudinal component E z is indeed an interesting issue. The simulated E z has a two-lobe transverse intensity profile, which is normalized to the on-axis intensity of E || . From their scale bars, the maximum intensity of two bright spots under E z is twice that of the spot under E || . Upon collection of an objective lens with a magnification of M , the intensity of optical field E z undergoes an M -fold reduction in amplitude to become E z / M at the imaging plane [44] , as shown in Fig. 3g . As a consequence, the amplitude of E z at the image plane has the order of 1/ M 2 (for example, 10 −4 in our experiment with M =100) of the actual E z at the objective plane. However, the transverse component of the electric field has no significant attenuation by the objective lens. That is why E z is usually negligible at the image plane of conventional optical imaging systems [44] . In fact, it is difficult to measure the E z component, which requires special techniques, such as utilizing tip-enhanced second-harmonic generation in scanning near-field optical microscopy [45] or using surface-enhanced Raman scattering [46] . It is important to emphasize that our FWHM is normalized to the wavelength in the same ambience (that is, air) throughout, instead of normalizing the FWHM observed in dielectric ambience (for example, oil) by the wavelength in air. In fact, the experimentally achieved 0.32 λ spot is much smaller than the super-oscillatory criterion ( r s =0.38 λ /numerical aperture (NA)) [43] , validating the physics of design to be in line with the super-oscillation phenomenon. This super-oscillatory spot requires the precise control of coherent interference of light from photon sieves, which means that our lens is more sensitive to chromatic aberration than traditional spherical lenses or other nanostructured lenses [14] , [15] , [16] , [17] that display larger spots. Although our photon sieve lens also suffers from low efficiency as other nanostructured lenses [14] , [15] , [16] , [17] , this technique is able to offer a direct and non-invasive way to realize super-resolution imaging without evanescent wave by incorporating it with scanning confocal microscopy [47] . It is worth commenting here that although in this reference the E-field at the focusing spot has an important longitudinal component, as in our case, the good imaging properties of the lens are preserved. Notice also that our approach has the advantage of sieving a single mode, as holes are used as DUs and not rings, as used in ref. 47 . Our approach could also be used to design various sophisticated optical sieving devices with randomness, and the currently reported lens is just one example showing the superfocusing performance. In addition, the proposed high-NA photon sieve with purely subwavelength-size units gets rid of the broken symmetry of the focusing spot, which usually occurs in subwavelength zone plates [16] . With its direct sub-diffraction limit focusing beyond the evanescent region in air ambient, ultrathin planar characteristics [48] and polarization insensitiveness, the photon sieve high-NA lens is promising to integrate with conventional imaging and focusing systems for optical micro-nanoscopy and nanolithography application. In summary, we have experimentally demonstrated the accurate manipulation of light beyond the evanescent region by using a random photon sieve to realize a uniform, twin-image free and high diffraction-efficiency hologram and a non-periodic photon sieve to focus light into a super-resolution spot with a size of 0.32 λ in air. Empowered by our hybrid approach to accomplish such a challenging design for devices carrying ultrahigh-capacity subwavelength unit elements, it opens up a new avenue to reach for multi-functionality nanophotonic devices with complex non-periodic structures. The hybrid approach for modelling far-field diffraction of subwavelength holes can be easily extended to apertures with any other regular shapes (for example, rectangle, ellipse, annulus and triangle). It is robust and universal for geometrical arrangement of unit elements to spatially manipulate amplitude, phase and polarization of light. The random photon sieve can find applications in integrated photonics and beam shaping owing to its polarization independence, ultrathin planarity, high field uniformity and high diffraction efficiency. The hybrid approach The hybrid approach can be implemented in two steps: (1) the coupled-mode theory is used to describe the electric field at the exit plane of a hole, and (2) the far-field diffraction of the electric field at the exit plane is described by the multipole expansion method. We briefly introduce the hybrid approach for the far-field diffraction of a nanoscale hole here. According to coupled-mode theory [3] , [22] , the electric field in the circular through hole (with radius a ) in a perfect electric conducting film with the thickness h can be expressed by the weighted superposition of the waveguide eigenmodes as follows: where − h ≤ z ≤0 with the hole’s entrance pupil at z =− h and exit pupil at z =0, α stands for one waveguide eigenmode, the modal electric field Ψ α ( r ′, ϕ ′) takes the form of Bessel function, as well as triangular function [49] , and the modal coefficient C α depends on the coupling between the incident light and the waveguide mode [22] . The modal coefficient C α for different z positions can be obtained by solving a linear matrix equation, which is related to the boundary conditions of electromagnetic field at the entrance and exit pupils, through the standard matrix-inversion technique [22] . In fact, one just needs the electric field E hole ( r ′, ϕ ′,0) at z =0. The far-field diffraction of a single hole can be regarded as the far-field radiation of induced source with its electric field E hole ( r ′, ϕ ′,0). In that case, we can use the superposition of multipoles to approximate the source because the far-field diffraction of multipole is a well-solved issue in classical electrodynamics [23] . Here, using the multipole expansion theory [23] , [24] , we show the electric field of the source E hole ( r ′, ϕ ′,0) as follows: where u is the unit vector u = r / r , r ′ is the position vector in the exit surface S ′ of the hole and n is the external normal vector detailed in Fig. 1a . Here we assume that the light illuminating the hole is a normally incident transverse electric (TE) (that is, y -polarized) plane wave so that only the vertically oriented TE and transverse magnetic (TM) waveguide modes (WGMs) are excited in the hole [22] . The vertically oriented modes are defined by Ψ α ( r ′, ϕ ′)=0.5· g nm {[ J n −1 ( χ nm r ′/ a )·sin( n −1) ϕ ′−(−1) s J n +1 ( χ nm r ′/ a )·sin( n +1) ϕ ′] e x ′ +[ J n− 1 ( χ nm r ′/ a )·cos( n −1) ϕ ′+(−1) s J n +1 ( χ nm r ′/ a )·cos( n +1) ϕ ′] e y ′ }, where g nm is the normalized constant of WGMs, J n (·) is the n th-order Bessel function of the first kind, χ nm is the factor determining the radial mode index and n and m are the azimuthal and radial mode indices, respectively. For the TE WGMs, s =1, χ nm is the m th non-nil zero of J ′ n ( x ) (the derivative of J n ( x )) and g nm =( e n /π) 1/2 χ nm /[ aJ n ( χ nm )( χ nm 2 − n 2 ) 1/2 ]; for the TM WGMs, s =0, χ nm is the m th non-nil zero of J n ( x ), g nm =( e n /π) 1/2 /[ aJ n −1 ( χ nm )], where e n is 2 except that e n =1 for n =0. After substituting E hole ( r ′, ϕ ′, 0 ) by the vertically oriented WGMs, one can find that equation (2) has the analytical solution in TE r.m.s. of Bessel functions where ρ 2 = x 2 + y 2 , r 2 = ρ 2 + z 2 , f n = a [ ηJ n−1 ( aη ) J n ( aɛ ) −ɛJ n−1 ( aɛ ) J n ( aη )]/( ɛ 2 −η 2 ), ɛ = χ nm / a , η = kρ / r . Equation (3) gives the analytical solution for the far-field diffraction of a single subwavelength hole, without any integral or differential formula involved. Far-field diffraction of nanosieve Subsequently, by using the coherent superposition of the diffracting field from every hole, we can get the far-field diffraction of the nanosieve where r′ j is the position of the j -th hole in a nanohole array and N is the total number of holes. We have to emphasize that the hole number N can be infinitely large according to practical requirement. Equation (4) is valid for the hole array with arbitrary distribution. Experimental setup The experimental measurement of the photon sieve hologram and superfocusing are carried out in a photon scanning tunnelling microscope (Alpha 300S, WITec GmbH) with confocal configuration, as shown in Figs 2b and 3b . A laser light with linear polarization is coupled to a polarization-maintaining single-mode fibre. To realize the plane wave incident on the photon sieve, a lens working as a collimator is located after the output terminal of the fibre. The collimated beam reflected by a mirror is normally incident on the fabricated photon sieve that is fixed on a three-dimensional computer-controlled stage. For photon sieve hologram under 532-nm-wavelength illumination, its transmitted light is collected by a × 10 magnification objective lens, whose position can be tuned by a high-precision stage along the propagating direction of light so that the objective lens can image the bird pattern onto a charge-coupled device camera directly. For photon sieve lens with NA≈0.83, its diffracting light is collected by a × 100-magnification objective lens with a higher NA of 0.9, so that the focused spot can be mapped without any distortion. A multi-mode fibre with a radius of 50 μm is located at the imaging plane of the objective lens for transferring the collected optical signals to the photomultiplier. The photomultiplier transforms the optical signal into an electric signal that can be detected by the same computer controlling the three-dimensional stage. The correlation between the three-dimensional stage position and the detected signal allows us to reconstruct a two-dimensional image of the diffracting field of photon sieve at a specified z-cut plane. How to cite this article : Huang, K. et al. Ultrahigh-capacity non-periodic photon sieves operating in visible light. Nat. Commun. 6:7059 doi: 10.1038/ncomms8059 (2015).